Biskyrmion states and their current-driven motion in a layered manganite The magnetic skyrmion is a topologically stable spin texture in which the constituent spins point to all the directions wrapping a sphere. Generation and control of nanometric magnetic skyrmions have large potential, for example, reduced power consumption, in spintronics device applications. Here we show the real-space observation of a biskyrmion, as defined by a molecular form of two bound skyrmions with the total topological charge of 2, realized under magnetic field applied normal to a thin plate of a bilayered manganite with centrosymmetric structure. In terms of a Lorentz transmission electron microscopy (TEM), we have observed a distorted-triangle lattice of biskyrmion crystal, each composed of two bound skyrmions with oppositely swirling spins (magnetic helicities). Furthermore, we demonstrate that these biskyrmions can be electrically driven with orders of magnitude lower current density (<10 8 A m −2 ) than that for the conventional ferromagnetic domain walls. There is increasing interest in nanometric topological spin textures in magnets, since they are expected to provide the means for electric control of magnetism. Among them, a skyrmion [1] , a nanometric spin-swirling vortex, is not only interesting for its unconventional electromagnetic actions but also promising for application to a new information bit [1] , [2] , [3] , [4] , [5] , [6] , [7] . The concept of skyrmion, originally introduced by Skyrme [8] as a model to describe a state of nucleon, is now extended to describe spin configurations in quantum Hall [9] and helimagnetic systems [1] , [10] , [11] , [12] . This particle-like nanometric magnetic object is topologically stable in a sense that this structure is not continuously transformed from conventional magnetic textures such as ferromagnetic (spin collinear) states. In the skyrmion, constituent spin directions can wrap a sphere, namely subtending a solid angle of 4π, as characterized by a topological charge (skyrmion number) of unity [1] , [11] , [12] , [13] . The topological charge or skyrmion number N s is defined as Here and M ( x , y ) represents the spatially in-plane varying local magnetization. Recent experimental observations have confirmed the theoretical prediction that skyrmions arise most typically from helical spin structures as generated by the relativistic spin antisymmetric exchange interaction, that is, Dzyaloshinskii–Moriya (DM) interaction [1] , [10] , [11] , [12] , [13] , [14] , [15] , [16] . In the single skyrmion, the magnetization curls in the inside and culminates along the out-of-plane direction in the core and periphery of the vortex; the direction of the core spins is opposite to that of the peripheral spins that are aligned along the applied magnetic field. As a spin-polarized electric current passes through the skyrmion, the moving electrons accept the fictitious Lorentz force induced by the topological charge (scalar spin chirality) from the curved spin texture of skyrmion. On the other hand, the skyrmions sense the counteracting Hall force [1] , [2] , [3] , [4] , [5] , [6] and spin transfer torque [17] , [18] , [19] to exhibit translational motions when the current exceeds some critical density for depinning [1] , [2] , [3] , [4] , [5] . Compared with the critical value for a drive of magnetic domain walls (MDWs) in ferromagnets, the threshold current density for that of skyrmions is extremely low since there is no intrinsic pinning effect on skyrmions [20] . Current-driven motion of skyrmions or skyrmion crystal (SkX) in the chiral-lattice magnets has been observed in recent experiments with an ultra-low current density, for example, five orders of magnitude smaller than that for a drive of MDWs [2] , [5] . This may present the first step towards the development of low power-consumption magnetic memory devices using skyrmions as information carriers [21] . In particular, increase of skyrmion density or skyrmion number may be useful to enhance the skyrmion transport toward high-density memory functions. The skyrmion formation has been observed not only for chiral-lattice magnets endowed with the DM interaction but also for centrosymmetirc magnets with uniaxial magnetic anisotropy, as exemplified by a recent observation of skyrmions with N s =1 in an M-type hexaferrite, BaFe 12− x −0.05 Sc x Mg 0.05 O 19 ( x =1.6) (ref. 22 ). In spite of the common topology, there are important differences between the skyrmions in the chiral-lattice and centrosymmetric-lattice systems. The first is the spin helicity degree of freedom; while the DM interaction in chiral-lattice magnets results in the unique spin-swirling direction (spin helicity) in skyrmions, the dipolar interaction in centrosymmetric ferromagnets induces two kinds of skyrmion states with opposite spin helicities. Second, the skyrmion size or skyrmion-crystal lattice constant depends strongly on sample thickness and external field in uniaxial ferromagnets [22] , in contrast to the fixed value as determined by the ratio of the symmetric exchange and DM interaction strengths in the chiral-lattice magnets [11] . Accordingly, the uniaxial ferromagnetic system provides a good arena to produce skyrmion textures with tunable size and spin helicity. We target here a ferromagnetic oxide, La 2−2 x Sr 1+2 x Mn 2 O 7 , which is known as a colossal magnetoresistance material showing a tetragonal layered structure ( I 4/ mmm ) with alternate stacking of magnetic conducting MnO 2 bilayers and non-magnetic insulating (La,Sr) 2 O 2 layers along the c axis [23] . The magnetic order and fluctuation give rise to a wealth of intricate magnetic configurations in the bilayer-structured manganite, such as spin-flip phenomenon and spontaneous bubble formation [24] , [25] . The magnetic easy axis varies with the hole concentration x , accompanying the spin-reorientation with changing temperature in 0.30 ≦ x <0.33 (ref. 26 ). The variety of magnetic structures has been accounted for in terms of the change of the relative occupancy in two e g orbital states (3 z 2 − r 2 and x 2 − y 2 ) (ref. 27 ). Here we report the experimental discovery of a nontrivial topological spin texture with a topological charge ( N s ) of 2, termed hereafter a biskyrmion, as produced by application of a magnetic field along the c axis on La 2−2 x Sr 1+2 x Mn 2 O 7 ( x =0.315). The observed biskyrmion is composed of two skyrmions with the opposite spin helicities and can be driven by a low current density of <10 8 A m −2 . 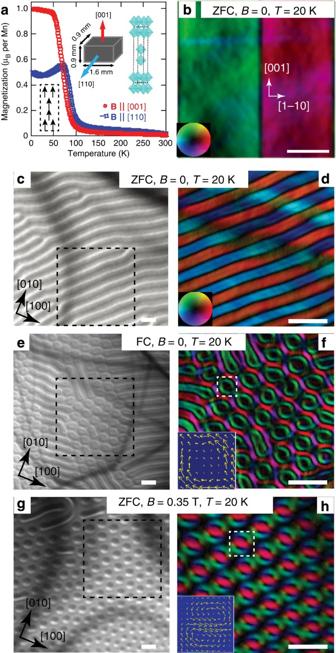Figure 1:Magnetic structures in a bilayered manganese oxide La2-2xSr1+2xMn2O7withx=0.315 and centrosymmetric space groupI4/mmm. (a) Temperature profiles of the in-plane and out-of-plane magnetizations at a magnetic field of 0.05 T applied along the [110] and [001] axes, respectively. Insets show the schematic illustration of bilayered perovskite structure (upper right panel), spin configuration (lower left corner) with uniaxial magnetic anisotropy below 60 K, and schematic drawing of a rectangular-shaped sample (middle) for magnetization measurements. (b) The ferromagnetic domains with out-of-plane magnetization represented by the lateral magnetization distribution as obtained by transport-of-intensity equation (TIE) analysis of the Lorentz transmission electron microscopy (TEM) data on the (110)-plane plate sample. (c,d) The under-focused Lorentz TEM image of in-plane spontaneous stripes (c) observed in the (001)-plane plate sample after zero field cooling (ZFC) and the corresponding spin texture (d) as obtained by TIE analysis of the Lorentz TEM data shown in the boxed area ofc. (e,f) The under-focused Lorentz TEM image (e) of magnetic bubbles and pinched-off stripes observed in the (001)-plane plate in zero field after the FC procedure in 0.15 T, and the corresponding spin texture (f) of the mixed magnetic structure shown in the boxed area ofe. (g,h) The under-focused Lorentz TEM image (g) in a magnetic field of 0.35 T applied normal to the (001)-plane plate at 20 K and the corresponding spin texture (h) of the biskyrmion lattice shown in the boxed area ofg. Insets tofandhshow the in-plane magnetization distributions of a bubble with a pair of Bloch lines and a biskyrmion in the boxed areas infandh, respectively. Scale bars inb–hcorrespond to 300 nm. Magnetic structure in La 2−2 x Sr 1+2 x Mn 2 O 7 with x =0.315 Figure 1 presents the temperature dependence of magnetization and the low-temperature spin textures in the x =0.315 compound. The crystal structure of the bilayer-structured manganite is schematically shown in the inset to Fig. 1a . The middle panel of the inset is a schematic drawing of a rectangular-shaped sample of 1.6 × 0.9 × 0.9 mm, in which the demagnetization coefficients are common as the applied magnetic field along [110] and [001] axes. Both in-plane and out-of-plane M–T curves ( Fig. 1a ) measured on this bulk crystal indicate the ferromagnetic transition temperature T C around 100 K and the magnetic easy axis along the [001] axis. A schematic of spin configuration is shown in the left corner of Fig. 1a . The uniaxial behaviour of the magnetic anisotropy was also clarified by the spontaneous magnetization textures of the (110)-plane and (001)-plane plate samples with the thickness of about 50 nm, as respectively shown in Fig. 1b,d , obtained by analysing Lorentz transmission electron microscopy (TEM) images using the transport-of-intensity equation (TIE). The colours mean the magnitude and direction of the lateral magnetizations, while dark colour indicates the magnetizations along the direction normal to the sample plate. Accordingly, the green and red coloured regions in Fig. 1b and the orange and blue coloured regions in Fig. 1d denote the antiparallel domains of magnetizations along the ‹001› axes and the ‹110› axes, respectively. The dark colours in Fig. 1b,d represent magnetizations along the ‹110› and the ‹001›, respectively, normal to the sample plates. The regular ferromagnetic domain structure with 180-degree MDWs (Bloch-type) in the (110) plane and the stripe domain structure (shown in Fig. 1c,d ) in the (001) plane manifest the uniaxial magnetic anisotropy for the compound. In particular, the regular stripe structure on the thin (001) plate ( Fig. 1d ) is formed by the magnetic dipolar interaction. According to the standard model by Garel and Doniach [28] , the application of a magnetic field normal to the thin plate is anticipated to change the stripes to the magnetic bubble lattice. Figure 1: Magnetic structures in a bilayered manganese oxide La 2-2x Sr 1+2x Mn 2 O 7 with x =0.315 and centrosymmetric space group I 4/ mmm . ( a ) Temperature profiles of the in-plane and out-of-plane magnetizations at a magnetic field of 0.05 T applied along the [110] and [001] axes, respectively. Insets show the schematic illustration of bilayered perovskite structure (upper right panel), spin configuration (lower left corner) with uniaxial magnetic anisotropy below 60 K, and schematic drawing of a rectangular-shaped sample (middle) for magnetization measurements. ( b ) The ferromagnetic domains with out-of-plane magnetization represented by the lateral magnetization distribution as obtained by transport-of-intensity equation (TIE) analysis of the Lorentz transmission electron microscopy (TEM) data on the (110)-plane plate sample. ( c , d ) The under-focused Lorentz TEM image of in-plane spontaneous stripes ( c ) observed in the (001)-plane plate sample after zero field cooling (ZFC) and the corresponding spin texture ( d ) as obtained by TIE analysis of the Lorentz TEM data shown in the boxed area of c . ( e , f ) The under-focused Lorentz TEM image ( e ) of magnetic bubbles and pinched-off stripes observed in the (001)-plane plate in zero field after the FC procedure in 0.15 T, and the corresponding spin texture ( f ) of the mixed magnetic structure shown in the boxed area of e . ( g , h ) The under-focused Lorentz TEM image ( g ) in a magnetic field of 0.35 T applied normal to the (001)-plane plate at 20 K and the corresponding spin texture ( h ) of the biskyrmion lattice shown in the boxed area of g . Insets to f and h show the in-plane magnetization distributions of a bubble with a pair of Bloch lines and a biskyrmion in the boxed areas in f and h , respectively. Scale bars in b – h correspond to 300 nm. Full size image Generation of a magnetic bubble lattice is observed in this compound even under zero magnetic field after 0.15 T field cooling (FC). Figure 1e shows the hexagonal bubble lattice accompanied by pinched-off stripes represented in an under focused Lorentz TEM image. The corresponding lateral spin textures are visualized in Fig. 1f , as obtained from TIE analyses of the Lorentz TEM data shown in the boxed region of Fig. 1e . It clearly reveals a mixed state with stripes (left region) and type II bubble lattice (center region) stemming from the pinched-off stripes; the bubble peripherals are composed of a pair of semicircular rings (non-monotone green) with the oppositely winding spins and the out-of-plane magnetization culminates at the core (see the magnified spin texture in the inset of Fig. 1f ). The respective bubbles on the triangular lattice are connected with each other by Bloch lines [22] , and hence their topological charge N s is zero. Thus such bubbles as accompanied by a pair of Bloch lines are topologically distinct from the skyrmions. Biskyrmion lattice formation and its spin texture The nontrivial spin texture with non-zero topological charge is observed ( Fig. 1g,h ) when a magnetic field (0.35 T) is applied to the stripe state along the c axis, that is, exactly normal to the (001)-plane plate (the orientation of the (001) thin plate was checked by the selected area electron diffraction pattern). Figure 1g is an under-focused Lorentz TEM image that represents distorted vortex-like magnetic configurations coexisting with minor isolated stripes with closed ends. The corresponding spin textures obtained by TIE analyses of Lorentz TEM data of highlighted portion of Fig. 1g are shown in Fig. 1h . The eight-figured topological spin textures form a distorted hexagonal lattice, which are distinct from both the single-helicity skyrmions in chiral magnets and the conventional magnetic bubbles with random spin helicities in ferromagnetic thin films. A magnified view of one unit of the distorted triangular lattice is displayed in Fig. 2a , and the lateral magnetization distributions are indicated with arrows in Fig. 2b . To scrutinize the spin texture of this eight-figured object, we show the bare Lorentz TEM images, under-focus ( Fig. 2c ) and over-focus ( Fig. 2d ), showing opposite magnetic contrasts. The TIE analysis ( Fig. 2e ) clearly shows that each spin texture is composed of two skyrmions with opposite magnetic helicities, that is, clockwise (CW) and counter-clockwise (CCW) spin curls. Although the Lorentz TEM cannot specify the direction (up or down) of the magnetization normal to the plate, the background black (that is, zero lateral component) parts in the core and the peripheral can be assigned to the upward and downward magnetizations (antiparallel and parallel to the applied field direction), respectively, considering that the net downward magnetization (parallel to the applied field) should remain finite. Therefore, this eight-figured magnetic object can be viewed as a bound state or a molecular form of two skyrmions with the same core spin directions (upward) and hence its topological charge should be twice of the single skyrmion number, that is, N s =2. On this ground, we call this spin vortex object biskyrmion . Here we can define the polarity of constituent skyrmions, plus (+) for the CW skyrmion and minus (−) for CCW skyrmion (that is, the magnetic helicity of spin texture). This polarity sign is identical with the toroidal moment sign of the skyrmion. The formation of biskyrmion stems from the helicity degree (+ or −) of freedom of each skyrmion, which can be realized only for centrosymmetiric magnets, not for chiral-lattice magnets with the DM interaction. If two skyrmions with the same helicity are brought together, the overlapping area would antiparallelly magnetize over a short distance, causing a strong increase in exchange energy. Contrary to this, if the helicity is different, the only moderate modification of spin orientation are necessary in the overlap region, making the CW and CCW composite state, that is, biskyrmion, relatively stable, as observed. 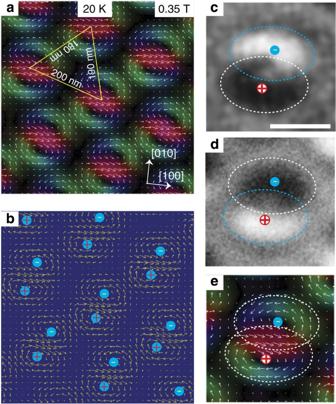Figure 2: Magnetic configurations of the biskyrmions. (a) The spin texture of biskyrmion lattice. (b) The in-plane magnetic component (yellow arrows) distribution in the biskyrmion lattice. (c,d) The over-focused (c) and under-focused (d) Lorentz TEM images for a biskyrmion. (e) The magnified view of spin texture for a biskyrmion. Inaande, colours and white arrows represent the magnitude and orientation of in-plane magnetizations, while the dark colour depicts the upward (downward) magnetizations in the core (periphery) of the biskyrmions. In (b–e), ‘plus’ (+) and ‘minus’ (−) indicate the magnetic helicity, that is, the clockwise and counter-clockwise rotating directions of in-plane magnetizations around the core, respectively. They are not the directions of magnetization along thezaxis. Scale bar inccorresponds to 100 nm. Figure 2: Magnetic configurations of the biskyrmions. ( a ) The spin texture of biskyrmion lattice. ( b ) The in-plane magnetic component (yellow arrows) distribution in the biskyrmion lattice. ( c , d ) The over-focused ( c ) and under-focused ( d ) Lorentz TEM images for a biskyrmion. ( e ) The magnified view of spin texture for a biskyrmion. In a and e , colours and white arrows represent the magnitude and orientation of in-plane magnetizations, while the dark colour depicts the upward (downward) magnetizations in the core (periphery) of the biskyrmions. In ( b – e ), ‘plus’ (+) and ‘minus’ (−) indicate the magnetic helicity, that is, the clockwise and counter-clockwise rotating directions of in-plane magnetizations around the core, respectively. They are not the directions of magnetization along the z axis. Scale bar in c corresponds to 100 nm. Full size image The biskyrmion triangular lattice shows an inequality regarding the sides that a ≠ b ≠ c , while the polar direction along the line connecting the two skyrmion cores or the skyrmionic molecular axis is fixed and one axis of the lattice side coincides with the pinched-off stripe direction (see Fig. 3a ). This is in contrast with the case of the random polarity (spin helicity) of skyrmions forming the hexagonal lattice observed in another centrosymmetric magnet, an M-type hexaferrite [22] . In other words, the interaction between the biskyrmions in this material is appreciable to form the ‘polar’ single domain of the biskyrmion crystal. 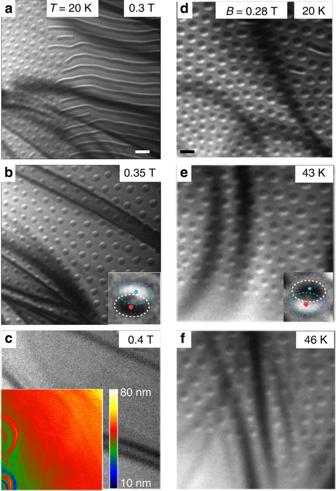Figure 3: Magnetic field and temperature dependence of biskyrmions in real-space Lorentz TEM images. (a–c) Magnetic field dependence of the magnetic configurations in real-space Lorentz TEM (over-focus) images at 20 K. (d–f) Temperature dependence of biskyrmions in Lorentz TEM (under-focused) images under a magnetic field of 0.28 T. Magnetic fields were applied normal to the (001) thin plate. The insets tobandeshow the enlarged view of a single biskyrmion. It should be noted that the bright and dark contrast is reversed inbandedue to the over- and under-focusing in the respective images. The colour image increpresents the thickness distribution of the view area ofa–f. Scale bars inaanddcorrespond to 300 nm. Figure 3: Magnetic field and temperature dependence of biskyrmions in real-space Lorentz TEM images. ( a – c ) Magnetic field dependence of the magnetic configurations in real-space Lorentz TEM (over-focus) images at 20 K. ( d – f ) Temperature dependence of biskyrmions in Lorentz TEM (under-focused) images under a magnetic field of 0.28 T. Magnetic fields were applied normal to the (001) thin plate. The insets to b and e show the enlarged view of a single biskyrmion. It should be noted that the bright and dark contrast is reversed in b and e due to the over- and under-focusing in the respective images. The colour image in c represents the thickness distribution of the view area of a – f . Scale bars in a and d correspond to 300 nm. Full size image Magnetic field and temperature dependence of biskyrmions The dynamical process of generation and annihilation of the biskyrmions was successfully observed by an in situ Lorentz TEM image movie (see Supplementary Movie 1 ), which was achieved with changing magnetic field from 0 to 0.4 T and then reducing to 0 T at 20 K. The movie demonstrates that the biskyrmion size strongly depends on the sample thickness and the external magnetic field. To show the dependence of the magnetic textures on the field-strength and the film thickness, we present in Fig. 3a–c the over-focused Lorentz TEM images of the (001) thin plate with a gradient in film thickness, taken at various magnetic fields applied normal to the plate at 20 K. Thickness map in the view area of the Fig. 3a–c is shown as an inset of Fig. 3c ; the minimal thickness is ~10 nm around the sample edge and sample thickness gradually increases in going away from the edge. The stripes appear to be pinched off and the distorted triangular biskyrmion lattice is dynamically induced in a field of 0.3 T ( Fig. 3a ) (see also Supplementary Movie 1 ). The distorted hexagonal biskyrmion lattice replaces the stripes ( Fig. 3b ) when the field exceeds 0.35 T. The biskyrmion size increases with the sample thickness and the field below a critical field and turn to shrink above the critical field. Then, biskyrmions completely disappear as the field exceeds 0.4 T ( Fig. 3c ). We have also observed that the biskyrmions accompanied by stripes are recreated as we gradually reduce the external magnetic field, and that they subsist even at B =0. Figure 3d–f shows the temperature dependence of the biskyrmions. The Lorentz TEM images (under focused images) were recorded in a constant perpendicular field of 0.28 T. The distorted hexagonal biskyrmion lattice is stabilized below 40 K and begins to melt at the thinner sample region above 40 K. When the temperature is above 60 K but yet lower than the ferromagnetic transition temperature ( T C ), no magnetic contrast is discerned. It is perhaps because the increase of temperature causes the flop of easy axis of magnetization, that is,, the spin-reorientation phenomenon, prior to reaching T C . Realization of biskyrmions in a microdevice As recently demonstrated experimentally [2] , [5] and theoretically [4] , [20] , an electrical current can drive the skyrmions in chiral-lattice DM magnets with ultra-low current density because of the deformable skyrmion spin texture and skyrmion-crystal lattice-form. Stimulated by these observations on the chiral-lattice magnets, for example, MnSi and FeGe, we attempted to manipulate biskyrmions in the present centrosymmetric magnet as well by passing an electric current. We fabricated a microdevice as schematically shown in Fig. 4a . 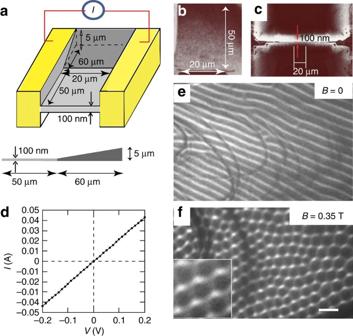Figure 4: Realization of biskyrmions in a microdevice. (a) Schematic of the device. (b,c) Scanning-ion-microscopy images of the plane and cross-section views of the device. (d)I–Vcurve for the device at 20 K. (e,f) The under focused Lorentz TEM images of the thinner region in the device under zero (e) and 0.35 T-field (f). The inset infshows the enlarged view of the biskyrmion lattice. Scale bar infcorresponds to 200 nm. Figure 4b,c presents the plane and cross-section views of the uniform La 2−2 x Sr 1+2 x Mn 2 O 7 ( x =0.315) thin plate in device, which was used for the electron beam transmittance. The characterization of electric current ( I ) versus voltage ( V ) shown in Fig. 4d indicates the ohmic contact between the electrodes and La 2−2 x Sr 1+2 x Mn 2 O 7 ( x =0.315) thin plate. We scrutinized the magnetic structure of the device before the current flows in the device. The stripy pattern (shown in Fig. 4e ) was observed under zero field and the distorted triangular biskyrmion lattice (shown in Fig. 4f ) was realized under a perpendicular magnetic field of 0.35 T. Figure 4: Realization of biskyrmions in a microdevice. ( a ) Schematic of the device. ( b , c ) Scanning-ion-microscopy images of the plane and cross-section views of the device. ( d ) I – V curve for the device at 20 K. ( e , f ) The under focused Lorentz TEM images of the thinner region in the device under zero ( e ) and 0.35 T-field ( f ). The inset in f shows the enlarged view of the biskyrmion lattice. Scale bar in f corresponds to 200 nm. 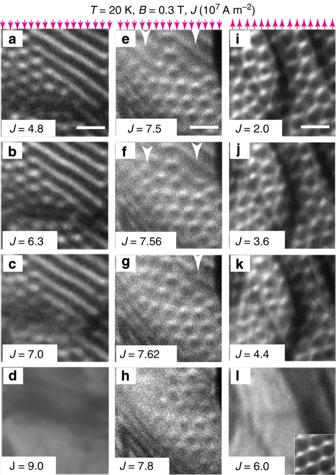Figure 5: Lorentz TEM images of stripes and biskyrmions obtained under current excitations. Changes in magnetic configurations with increasing currentJ(in unit of 107A m−2), obtained under a magnetic field of 0.3 T applied normal to the (001)-plane device plate at 20 K. (a–d) A mixed state of screws and biskyrmions atJ=4.8–9.0 × 107A m−2,e–ha mixed state at finely tunedJ(=7.5–7.8 × 107A m−2) and (i–l) a single-phase biskyrmion lattice state atJ=2.0–6.0 × 107A m−2. Red arrows indicate the current direction. The inset at the right bottom corner shows the biskyrmion lattice without current excitation. Scale bars ina,eandicorrespond to 500 nm. Full size image Current-driven biskyrmion motion in a mixed state Figure 5 shows changes in magnetic configurations with electric currents in the microdevice. The images in Fig. 5 were extracted from Supplementary Movies 2–4 , which were recorded by in-situ Lorentz TEM observations while passing current across the device at 20 K (the detailed information for Supplementary Movies 2–4 is described in the captions of Supplementary Movies ). As the current passes through the device at zero magnetic field, no significant change occurs for the spontaneous stripes (see Supplementary Movie 5 ), ensuring that the joule heat induced by such a low current density should not increase the device temperature above the T C . When we applied a magnetic field of 0.3 T on the device, the biskyrmions began to be generated in the thinner region of the device (see Fig. 4f ). First, we passed current, the direction of which is shown by red arrows in Fig. 5 , through a mixed state of biskyrmion lattice and stripe. The in situ Lorentz TEM images ( Fig. 5a–d ) show that the biskyrmions appear to flow, that is, become undiscerned in the still picture, under the current excitations above J =7.0 × 10 7 A m −2 , while the stripe is kept intact. It is to be noted here that the dynamical motion of biskyrmions cannot be captured directly because of much slower frame rate (1 frame per second) as compared with the skyrmion motion [5] and hence shows up as suddenly blurred skyrmion images. In contrast to the robust spontaneous ( B =0) stripes below current density of 2.52 × 10 8 A m −2 (see the Supplementary Movie 5 ), the stripes in the mixed state at B =0.3 T become undiscerned as well as the biskyrmions upon the current excitation above 9.0 × 10 7 A m −2 (see Fig. 5d ). Figure 5: Lorentz TEM images of stripes and biskyrmions obtained under current excitations. Changes in magnetic configurations with increasing current J (in unit of 10 7 A m −2 ), obtained under a magnetic field of 0.3 T applied normal to the (001)-plane device plate at 20 K. ( a – d ) A mixed state of screws and biskyrmions at J =4.8–9.0 × 10 7 A m −2 , e – h a mixed state at finely tuned J (=7.5–7.8 × 10 7 A m −2 ) and ( i – l ) a single-phase biskyrmion lattice state at J =2.0–6.0 × 10 7 A m −2 . Red arrows indicate the current direction. The inset at the right bottom corner shows the biskyrmion lattice without current excitation. Scale bars in a , e and i correspond to 500 nm. Full size image Current triggers transformation from stripes to biskyrmions To scrutinize the critical motion of stripes in coexistence with biskyrmion lattice, we have captured the Lorentz TEM images by finely varying the current immediately above the current density of 7.5 × 10 7 A m −2 . Figure 5e–h clearly evidences a metamorphosis of stripes (spin screw state) to biskyrmions in the critical current region. When the current is <7.5 × 10 7 A m −2 , the curved stripes accompanied by biskyrmions (white arrows in Fig. 5e–g ) are discerned in Fig. 5e . With further increasing current up to 7.56 × 10 7 A m −2 , as shown in Fig. 5f , the stripes begin to undergo fragmentation and partially transform to biskyrmions. As the current density is increased above 7.62 × 10 7 A m −2 , the stripes transform completely to biskyrmions (see Fig. 5g ), which eventually start to flow as seen in Fig. 5h . Thus the electric current can trigger the dynamical transformation from stripes to biskyrmions in some critical region of external magnetic field and temperature, where the biskyrmions and stripes can coexist due to their first-order transition nature. Current-driven biskyrmion motion in biskyrmion state Next we show the change of the biskyrmion lattice single phase under the excitation of current ( Fig. 5i–l ). A series of in situ Lorentz TEM images observed with increasing the current density display the overall motion of the biskyrmion lattice. Compared with the biskyrmion lattice without current, the individual biskyrmions ( Fig. 5i ) appear to be deformed (elongated) in shape at a lower current density of 2.0 × 10 7 A m −2 . The further increase in the current density up to 4.4 × 10 7 A m −2 appears to decrease the biskyrmion size, while the partial lattice appears to be subject to flow (that is, disappearing in the time-averaged image). Finally, all of the biskyrmions flow away at the current density above 6.0 × 10 7 A m −2 , which is lower than that for driving the biskyrmions in case of their coexistence with stripes. We have found biskyrmions with topological charge of 2 in a thin plate of a bilayer-structured manganite with uniaxial magnetic anisotropy. Each biskyrmion shows up as a bound state of two skyrmions with opposite magnetic helicities, and by gathering they form the distorted triangular lattice. Under current excitations, the screw state (stripe) coexisting with the biskyrmion is turned to the biskyrmions and then eventually the biskyrmions can flow. The critical current for driving biskyrmions is 2 orders higher than that for skyrmions in chiral-lattice magnets, MnSi (ref. 2 ) and FeGe (ref. 5 ), yet still 2–5 orders of magnitude lower than that for driving MDWs in ferromagnetic semiconductors [29] and alloys [30] . Compared with the single skyrmion in chiral-lattice magnet, the topological charge and the size of skyrmion in the centrosymmetric magnet are easily controlled by the sample geometry and external field or electrical current owing to its metastable nature. In addition, the doubled topological charge in the biskyrmion may cause a difference in the dynamics and also modify the skyrmion transport properties compared with the case of the single skyrmion, which remains to be investigated in future. Thus, such nanometer-scale biskyrmions or skyrmions in ubiquitous centrosymmetric magnets are also a potential candidate of electrically controllable information carrier in spintronics. Characterization of magnetic structure of biskyrmion A single crystal of La 2−2 x Sr 1+2 x Mn 2 O 7 ( x =0.315) was grown by the floating zone method. The thin plates were cut from bulk and thinned by mechanical polishing and argon ion milling. The crystal structure, magnetic configuration and the thicknesses of thin samples were measured by using the conventional TEM, Lorentz TEM and the electron energy loss spectroscopy (EELS), respectively. By using Lorentz TEM, the MDWs can be imaged as converges (bright contrast) or diverges (dark contrast) of the electron beam on the defocused (under- or over-focused) image planes. The inversion of such magnetic contrast can be seen between the over- and under-focused images [31] . To perform the quantitative in-plane magnetizations in Lorentz TEM configurations, TIE [32] was adopted with use of a software package QPt [33] . Preparation and characterization of a microdevice Current-driven biskyrmion motion were carried out using a microdevice made up of La 2−2 x Sr 1+2 x Mn 2 O 7 ( x =0.315) trapezoidal plate and two electrical conducting blocks at two sides of the plate. The trapezoid-shaped (001) plate of 20 μm × 110 μm × t (thickness: 100 nm–5 μm) was fabricated by a focused-ion-beam (FIB) instrument (Hitachi FB-2100) equipped with gallium ion gun. The electric conducting layer (a ~100-nm-thick Au-Pd polycrystalline film) was deposited on the device. From the scanning-ion-microscopy (SIM) measurement of the sample size we estimated that the electric current density is ~6.0 × 10 6 Am −2 as a current of 1 mA passes through the device. The dc current was supplied by a source–measure unit instrument (Keithley 2612A). How to cite this article: Yu, X. Z. et al. Biskyrmion states and their current-driven motion in a layered manganite. Nat. Commun. 5:3198 doi: 10.1038/ncomms4198 (2014).